Single-molecule electroluminescence and photoluminescence of polyfluorene unveils the photophysics behind the green emission band Optoelectronic properties of polyfluorene, a blue light-emitting organic semiconductor, are often degraded by the presence of green emission that originates mainly from oxidation of the polymer. Here, we use single-molecule electroluminescence (EL) and photoluminescence (PL) spectroscopy on polyfluorene chains confined in vertical cylinders of a phase-separated block copolymer to spectrally resolve the green band and investigate in detail the photophysical processes responsible for its appearance. In both EL and PL, a substantial fraction of polyfluorene chains shows spectrally stable green emission which is ascribed to a keto defect. In addition, in EL, we observe a new type of vibrationally resolved spectra distributed over a wide range of frequencies and showing strong spectral dynamics. Based on quantum chemical calculations, this type is proposed to originate from charge-assisted formation and stabilization of ground-state aggregates. The results are expected to have broad implications in the fields of photophysics and material design of polyfluorene materials. Polyfluorenes are a class of semiconducting π-conjugated polymers with excellent optical, electrical and mechanical properties that make them suitable for applications in optoelectronic devices [1] , [2] , [3] , such as organic light-emitting diodes (OLED) and related display and lightning technology [4] , [5] . Polyfluorenes are used as light-emitting and charge-transporting materials because of their pure blue color and high quantum efficiency of luminescence in solid state, high-charge mobility, good solubility and easy processability. However, light emission of polyfluorenes often shows an undesirable feature, an additional emission band in the green spectral region (a green band), which degrades the color purity and decreases the device efficiency and stability. The green band can appear both in photoluminescence (PL) and electroluminescence (EL) of thin films as a result of thermal treatment and is generally more pronounced in EL [2] . Over the past decade, great effort has been spent to clarify its origin and to devise ways to suppress the unwanted emission. Technologically, the problem can be solved by suitable material design [6] and device fabrication technology. In the initial studies, the origin of the green band has been ascribed to the formation of excited state aggregates, excimers [7] , [8] . Excimers have been known to form in concentrated solutions of fluorene monomers [9] as well as of polyfluorenes [10] . Arguments supporting the excimer origin came from the observations that the green band in emission of solid films is suppressed by restricting the polymer chain mobility or interchain interactions, for example, by introducing different chromophores in the main chain [11] or as side groups [12] , [13] , by mixing polyfluorenes with polymers of higher glass transition temperature [14] or by cross-linking the main chains [15] . Later, however, it has been shown that emission in the green spectral range originates from a keto defect formed as a result of photooxidation or thermal oxidation [16] , [17] , [18] , [19] , [20] , [21] , [22] . Copolymers and oligomers containing well-defined fractions of fluorenone as a model of the oxidized species showed emission from the fluorenone unit that is photophysically identical to the green band in polyfluorene [23] . Some studies indicated that interchain interactions between fluorenones and formation of excimers are required for the appearance of the green band [24] . These claims have later been disputed by single-chain spectroscopic experiments [25] . The prevalence of the green band in EL can be explained by assuming that charges are preferentially trapped on low-energy sites in the film, the fluorenone defects. Charge recombination on these low-energy sites gives rise to the green emission in EL. Although there is undoubtable evidence that oxidative defects in polyfluorenes are responsible for the substantial part of the green emission, the overall picture can be more complex and involve other photophysical mechanisms. Part of the reason that there has not been a clear consensus on the topic is that the amorphous polyfluorene films are heterogeneous systems, and conventional spectroscopic and other characterization methods provide only bulk-averaged values. Single-molecule spectroscopy is known as an effective method that removes the ensemble averaging and has been successfully used in studies of polymers and other complex soft matter [26] , [27] , [28] , including the observation of electrically induced chemiluminescence from single conjugated polymer nanoparticles [29] . In particular, it is the ability of single-molecule spectroscopy to reveal static distributions in spectra of individual molecules (inhomogeneous broadening) and temporal spectral changes (spectral diffusion) that make it well suited for the study of the inhomogeneous green band. Here, we report EL and PL spectroscopy on single-polyfluorene chains. We spectrally resolved the green emission band and investigated differences in the related photophysical properties between the EL and PL processes. Detection of EL from single chains of a conjugated polymer is made possible by isolating individual polyfluorene chains in vertical cylinders of a phase-separated block copolymer (BC), which is used as an emitting layer in an OLED device. In EL, we observed two types of single-chain spectra within the region of the green band, a vibrationally resolved short-wavelength type I and a broad structureless long wavelength type II, as well as strong spectral dynamics. In PL, only the long wavelength type II is present. The so far unknown type I is inconsistent with the keto defect emission. Based on quantum chemical calculations, we assign this type to emission from a ground-state dimer, which is formed and stabilized by a charge-assisted mechanism in the current-carrying OLED device. Doped BC films as active layers in OLED The polyfluorene used is poly[9,9-bis(3,6-dioxaheptyl)-fluorene-2,7-diyl] [7] (BDOH-PF, Fig. 1a ). The 3,6-dioxaheptyl sidechains in the BDOH-PF are short oligomers of poly(ethylene oxide) (PEO), which is a hydrophilic polymer. To stretch individual BDOH-PF chains between two electrodes in an OLED device and to immobilize them in an optically and electrically inert environment, we made use of a phase-separated BC, PEO m -b-PMA(Chal) n ( Fig. 1a ). The amphiphilic BC consists of a PEO block and of a hydrophobic block of polymethacrylate with chalcone mesogen in the side chains (PMA(Chal)) [30] . An annealed BC film forms hexagonally arranged PEO cylinders that span continuously the whole-film thickness. Thermodynamically, the PEO domains are in liquid phase at room temperature. The PEO sidechains of BDOH-PF ensure that the polymer mixes with the PEO phase ( Supplementary Fig. 1 ) of the BC and on annealing of a mixed spin-coated film the BDOH-PF chains are confined in the vertical cylinders of the BC film [31] ( Fig. 1b ). Transmission electron microscopy ( Fig. 1c ) and atomic force microscopy ( Fig. 1d ) of a 70 nm thick BC film doped with on average 1 BDOH-PF chain per cylinder reveal average cylinder diameter of 13 nm and cylinder-to-cylinder distance of 33 nm, as expected for this type of BC [30] . PL spectra of BDOH-PF in the BC are almost identical to those of BDOH-PF dispersed in a PEO homopolymer film ( Fig. 1e ). The spectra consist of a 0–0 band at 428 nm, a vibrational progression and broad emission in the long wavelength part, the green band. 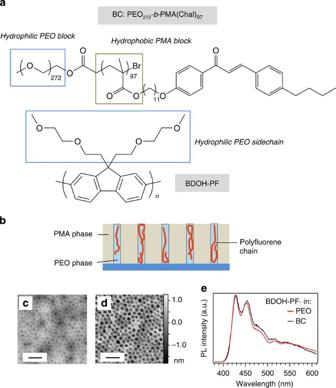Figure 1: Materials and characterization of the doped BC films. (a) Structure of the BC and of the polyfluorene BDOH-PF. (b) Scheme of the doped BC film. (c) Transmission electron microscopy image and (d) atomic force microscopy image of a BC film doped with BDOH-PF at the concentration of one chain per cylinder. Scale bars, 100 nm. (e) PL spectra of BDOH-PF doped in BC (black) and dispersed in a film of PEO homopolymer (red). Figure 1: Materials and characterization of the doped BC films. ( a ) Structure of the BC and of the polyfluorene BDOH-PF. ( b ) Scheme of the doped BC film. ( c ) Transmission electron microscopy image and ( d ) atomic force microscopy image of a BC film doped with BDOH-PF at the concentration of one chain per cylinder. Scale bars, 100 nm. ( e ) PL spectra of BDOH-PF doped in BC (black) and dispersed in a film of PEO homopolymer (red). Full size image The BDOH-PF-doped BC film is used as the active layer in an OLED device consisting of an Al cathode (100 nm), poly(3,4-ethylenedioxythiophene) polystyrene-sulphonate (PEDOT:PSS) hole-injection layer (40 nm) and indium–tin oxide (ITO) anode (56 nm) on a microscope cover glass ( Fig. 2a ). A device prepared with the doping concentration of one BDOH-PF chain per cylinder showed onset of emission at 5 V and maximum luminance of 1 cd m −2 ( Supplementary Fig. 2a ). The microscopic EL image in Supplementary Fig. 2b reveals spatial heterogeneity of EL intensity that is typical for conjugated polymer devices. A control device made with an undoped BC film containing only the vertical PEO cylinders also shows EL emission but the device is less stable, the onset voltage is at 13 V (compared with the 5 V of the doped device above) and the maximum luminance is two orders of magnitude lower ( Supplementary Fig. 2a ). Experiments on other control devices using an active layer of PEO homopolymer doped with different concentrations of BDOH-PF ( Supplementary Fig. 2c ) show that states resulting from interactions between the PEO and BDOH-PF do not contribute to the observed EL, and that the presence of the cylinders is crucial for the EL operation for devices with concentrations of BDOH-PF below 10 −8 M. These observations strongly support the assignment of the EL observed from the BC cylinders to the emission of the BDOH-PF chains ( Supplementary Note 1 ). 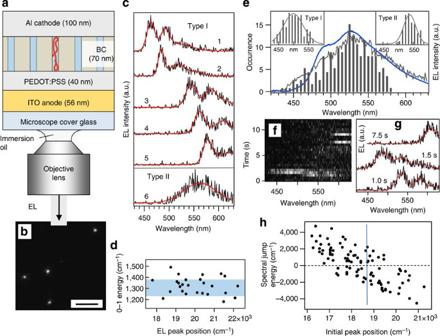Figure 2: Single-molecule EL. (a) Device structure of the OLED for single-molecule EL spectroscopy. (b) Microscopic image of EL from a device with BC film doped with BDOH-PF at the concentration of one chain per 100 cylinders taken at 8 V. Scale bar, 5 μm. (c) EL spectra from individual spots in the EL image taken at 8 V and integrated for 0.5 s. (d) Energy difference between the 0–0 and 0–1 bands of vibrationally resolved single-molecule EL spectra plotted as a function of the 0–0 band position. (e) Histogram of the peak positions of single-molecule EL spectra of 202 molecules (grey bars), together with a bulk EL spectrum of a control device prepared with a neat film instead of the BC (blue line) and with a sum of EL spectra of 70 single BDOH-PF molecules (grey line). Insets show histograms of the type I (left) and type II (right) spectral peak positions. (f) Example of EL spectral time evolution of one BDOH-PF molecule. (g) Examples of single-molecule EL spectra taken at three different times fromf. (h) EL spectral jump energy (energy after jump minus energy before jump) as a function of the initial peak position before the jump. Figure 2: Single-molecule EL. ( a ) Device structure of the OLED for single-molecule EL spectroscopy. ( b ) Microscopic image of EL from a device with BC film doped with BDOH-PF at the concentration of one chain per 100 cylinders taken at 8 V. Scale bar, 5 μm. ( c ) EL spectra from individual spots in the EL image taken at 8 V and integrated for 0.5 s. ( d ) Energy difference between the 0–0 and 0–1 bands of vibrationally resolved single-molecule EL spectra plotted as a function of the 0–0 band position. ( e ) Histogram of the peak positions of single-molecule EL spectra of 202 molecules (grey bars), together with a bulk EL spectrum of a control device prepared with a neat film instead of the BC (blue line) and with a sum of EL spectra of 70 single BDOH-PF molecules (grey line). Insets show histograms of the type I (left) and type II (right) spectral peak positions. ( f ) Example of EL spectral time evolution of one BDOH-PF molecule. ( g ) Examples of single-molecule EL spectra taken at three different times from f . ( h ) EL spectral jump energy (energy after jump minus energy before jump) as a function of the initial peak position before the jump. Full size image Single-molecule EL For single-molecule spectroscopy, the doping concentration was lowered to one BDOH-PF chain per 100 cylinders. Under such conditions, the EL image shows several isolated emission spots ( Fig. 2b ). Although the emission from individual spots is fluctuating in time (blinking, as described in detail below), the device itself continued stable EL emission for hours of the duration of the experiments. Fresh devices were prepared for new experimental days and the data taken on different days were fully reproducible. The EL spectra measured from individual spots can be divided into two types—narrow vibrationally resolved type I (spectra 1–5 in Fig. 2c ) and broad structureless type II (spectrum 6 in Fig. 2c ). The energy difference between the 0–0 and 0–1 vibrational bands in type I is constant over the range of spectral peak positions observed ( Fig. 2d ) and corresponds approximately to the energy of C–C inter-ring stretching in polyfluorenes [32] . Histogram of single-molecule EL spectral peak positions plotted for 202 molecules in Fig. 2e indicates a broad distribution stretching from 438 nm to 588 nm. The shape of the histogram reflects well a bulk EL spectrum (blue line in Fig. 2e ) measured on a reference OLED device with a neat homopolymer film as the active layer. In addition, the Fig. 2e shows as a grey line a sum of 70 EL spectra of single BDOH-PF molecules. The sum EL spectrum also agrees well with the bulk reference EL spectrum, especially in the onset and tail parts. Both the histogram and the sum spectrum, as well as the bulk EL spectrum show an absence of the 428 nm spectral band, which is dominant in PL. The bulk EL spectrum has a peak at 526 nm with a shoulder at 490 nm, and the green band dominates the emission. The shape of the spectrum is identical to that reported before for BDOH-PF [33] . The insets of Fig. 2e show results of sub-classification of the spectral peak distribution into the spectral types I and II. The histogram of the type I (left) is centered at 499 nm, the type II (right) has center at 538 nm. The spectra are distributed almost evenly between the two types, with 52% belonging to the type I and 48% to the type II. The EL from most of the individual spots is dynamic. The EL intensity undergoes blinking which is often accompanied by spectral changes (jumps), as seen in Fig. 2f,g , and in Supplementary Fig. 3a–f . The jumps occur both to the red and blue part of the spectrum. Also, the jumps can be between the two spectral types as well as within the same type ( Fig. 2g ). Overall, 71 out of the 202 molecules detected (that is, 35%) showed spectral jumps. The energy of the jumps is widely distributed and is correlated with the initial spectral position before the jump ( Fig. 2h ). In Fig. 2h , positive energy values correspond to red shift jump, negative values to blue shift jump. The correlation indicates that the further the initial spectral position of the molecule is from an apparent equilibrium the larger the spectral jump. The jump tends to return the molecule to that equilibrium. From the above experiments, we do not have direct evidence that the emission of individual spots comes from single BDOH-PF chains. However, the observed photophysical behavior (emission blinking, spectral distribution and spectral jumps) indicates that the EL originates from a single quantum emitter, which can be physically located on a single chain or on an aggregate of a few short chains. For the purpose of the present study and the implications of the results, the difference between a single chain and a small aggregate of short chains, which means the presence or absence of a few conjugated bonds can be neglected. Single-molecule PL The single-molecule EL experiments were further reproduced in PL on single chains of BDOH-PF dispersed in a thin film of PEO homopolymer ( Fig. 3a ). The majority of single molecules show spectra with well-resolved vibrational structure and 0–0 peaks between 420 and 430 nm (spectrum 1 of Fig. 3b ). This type of spectra can be assigned to the emission of a singlet exciton of an isolated polyfluorene chain (SE type). Large fraction of the molecules also showed spectra (such as spectrum 2 in Fig. 3b ), which correspond in shape and spectral range to the type II observed in EL. Occasionally, both the SE and type II appear together in a spectrum of one molecule (spectrum 3 of Fig. 3b ). On rare occasions, we also observed spectra (no. 4 and 5 of Fig. 3b ), which are located in the same spectral region as the type I in EL but have less pronounced vibrational structure. Histogram of spectral peaks of 216 molecules ( Fig. 3c ) shows a narrow distribution centered at 424.6 nm (SE type), which reflects well the 0–0 band of a bulk spectrum obtained on a PEO film doped with ensemble-level concentration of BDOH-PF ( Fig. 3c , blue line). In addition, the histogram shows a broad distribution (enlarged in the inset) centered at 537.8 nm of the type II spectra. Of the 216 molecules observed, 71% are of the SE type, 24% of the type II and the remaining 5% are located in the spectral region of type I. 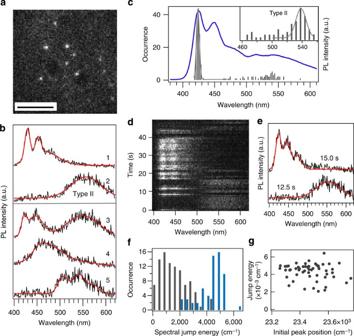Figure 3: Single-molecule PL. (a) Microscopic PL image of a PEO film doped with BDOH-PF at the concentration of 10−11M. Scale bar, 5 μm. (b) PL spectral from individual spots in the PL image integrated for 0.5 s. (c) Histogram of the peak positions of single-molecule PL spectra of 216 molecules together with a bulk PL spectrum of a control sample prepared with an ensemble-level concentration of BDOH-PF (blue line). Insets show detailed histogram of the type II spectral peak positions. (d) Example of PL spectral time evolution of one BDOH-PF molecule. (e) Examples of single-molecule PL spectra taken at two different times fromd. (f) Histogram of absolute values of spectral energy jumps for EL (grey) and PL (blue). (g) PL spectral jump energy (energy after jump minus energy before jump) as a function of the initial peak position before the jump. Figure 3: Single-molecule PL. ( a ) Microscopic PL image of a PEO film doped with BDOH-PF at the concentration of 10 −11 M. Scale bar, 5 μm. ( b ) PL spectral from individual spots in the PL image integrated for 0.5 s. ( c ) Histogram of the peak positions of single-molecule PL spectra of 216 molecules together with a bulk PL spectrum of a control sample prepared with an ensemble-level concentration of BDOH-PF (blue line). Insets show detailed histogram of the type II spectral peak positions. ( d ) Example of PL spectral time evolution of one BDOH-PF molecule. ( e ) Examples of single-molecule PL spectra taken at two different times from d . ( f ) Histogram of absolute values of spectral energy jumps for EL (grey) and PL (blue). ( g ) PL spectral jump energy (energy after jump minus energy before jump) as a function of the initial peak position before the jump. Full size image Similar to EL, 29% of the single BDOH-PF chains show spectral jumps. In PL, the jumps occur almost exclusively between the SE type and type II ( Fig. 3d,e ; Supplementary Fig. 4a ). Both the SE and type II can coexist in the spectra for part ( Supplementary Fig. 4b ) or all ( Supplementary Fig. 4c ) of the measurement interval. The spectra corresponding to the type I region appear during the jumps very rarely and only for a short period of time ( Supplementary Fig. 4d,e ). Compared with the EL that shows a broad range of jump energies (grey bars in Fig. 3f ), the jump energy in PL has a narrow distribution centered at 4,690 cm −1 (blue bars in Fig. 3f ) and the energy does not depend on the initial peak position of the spectra ( Fig. 3g ). In the above experiments, a common feature in both EL and PL is the presence of the type II spectra. A considerable fraction of the single chains showed spectrally stable emission of this type throughout the observation interval (examples are shown in Supplementary Fig. 3g,h for EL and in Supplementary Fig. 4c for PL). In terms of the spectral shape and distribution of spectral peaks, this type II is consistent with the emission from the keto defect (fluorenone emission). This assignment is supported by previous single-molecule studies of a model system containing a fluorenone emitter, which revealed structureless single-molecule spectra and a distribution of spectral peaks centered at 540 nm [34] , similar to the distributions observed here for type II in both EL and PL. In addition to the stable emission of type II (the keto defect), we observed notable differences in the spectral properties between EL and PL. The main difference of EL compared with PL is the absence of the SE type and the considerable contribution of the type I spectra. In terms of spectral shape and wavelength range, the type I cannot originate from either the fluorenone or excimer emission, because these are invariably characterized by broad structureless lineshapes. In general, planarization of the polyfluorene main chain (formation of β-phase) leads to extension of the π-conjugation length and to red-shifted vibrationally resolved absorption and emission spectra [3] , [35] . However, the red shift of β-phase has never been observed to stretch into the spectral region of the type I and, thus, the main chain planarization can also be excluded as the origin of this type of spectra [36] . Other possible explanations of the type I might include delayed fluorescence of phosphorescence. However, as also shown in literature, delayed fluorescence is spectrally identical to prompt fluorescence [36] . Phosphorescence is observable only at cryogenic temperatures [36] and its rate (~1 s −1 ) would preclude observation on single-molecule level. Here, based on density functional theory (DFT) calculations, we propose a charge-assisted formation and stabilization of ground-state dimers as the origin of the type I spectra in EL. The DFT calculations show that neutral monomer fluorene molecules can form stable van der Waals dimers with an average binding energy of −49.6 kJ mol −1 ( Supplementary Fig. 5 ; Supplementary Table 1 ). A calculated first excited state energy (HOMO-LUMO gap) of the dimer results only in a few nanometre shift of the optical transition energy with respect to a monomer ( Supplementary Table 2 ) and the dimer is not observable in absorption spectra. Due to computational reasons, the bulk of the calculations were performed on fluorene with methyl groups at the 9,9 positions. We have verified on selected examples that replacement of the methyl groups with ethylene oxide does not affect the observed phenomena ( Supplementary Fig. 6 ). Fluorenes with the ethylene oxide side groups do form both neutral and mixed dimers and the binding energy in most cases further increases compared with the methyl-substituted fluorenes ( Supplementary Table 3 ). 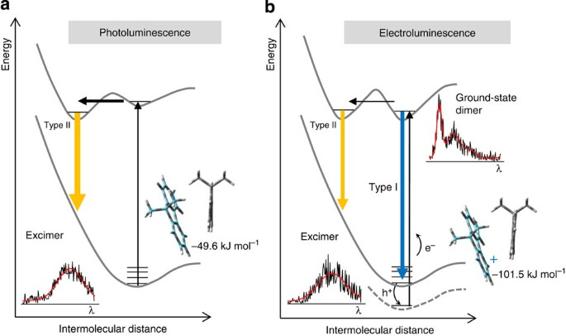Figure 4: Scheme of the proposed energy levels and the optical transitions. (a) PL. (b) EL. In the EL scheme, the neutral ground-state dimer is stabilized by the injection of a charge (for example, a hole h+). Recombination with the opposite charge (an electron e−) leads to the population of a neutral dimer excited state in a configuration corresponding initially to the mixed dimer ground state before recombination. The molecular orbital properties and interorbital transitions are also similar to the methyl-substituted fluorenes ( Supplementary Table 4 ). To explain the spectral dynamics and spectral type changes in both PL and EL, we first put forward a model that involves excimer emission. We assume that in PL, on excitation, the ground-state dimers transform into excimers ( Fig. 4a ) and emit spectra that are similar to the type II. This transformation process has been experimentally observed on fluorene monomers in supersonic jets [37] . The excimer state has lower potential energy and the inter-molecular distance in the excimer is shorter than that in the corresponding excited state of the dimer. The excimer decays radiatively into a ground-state configuration, which does not have a potential minimum and this configuration transforms again into the ground state of the dimer. In condensed state, similar formation of excimers has been observed in the emission of molecular crystals, which themselves are a form of ground-state aggregates [38] and in conjugated polymers where the primary excitation is also a singlet exciton which rapidly transforms into an excimer state [39] . The spectral jumps between the SE and type II spectra result likely from local conformational changes of the BDOH-PF chains between states that allow the formation of the ground-state aggregates and states in which the distance between the neighboring chains is such that the aggregates do not form and the emission comes from singlet excitons on isolated chains. Figure 4: Scheme of the proposed energy levels and the optical transitions. ( a ) PL. ( b ) EL. In the EL scheme, the neutral ground-state dimer is stabilized by the injection of a charge (for example, a hole h + ). Recombination with the opposite charge (an electron e − ) leads to the population of a neutral dimer excited state in a configuration corresponding initially to the mixed dimer ground state before recombination. Full size image The excitation process in EL involves injection and trapping of charges on the fluorene units. This is followed by charge recombination when an opposite charge arrives at the molecule. To simulate such situation, we carried out the DFT calculations on a mixed dimer formed between a neutral fluorene monomer and a fluorene cation or anion. The calculations reveal ( Supplementary Table 1 ) that the binding energy is much larger for the mixed dimer of a neutral monomer and a cation (average binding energy of −101.5 kJ mol −1 ) as well as anion (average binding energy of −84.8 kJ mol −1 ). The averages are means of the values from Supplementary Table 1 . Such further stabilization of the ground state by charge trapping leads to a more efficient formation of the mixed dimer from the monomers and to the complete absence of the SE type emission in EL. The stabilization occurs also in the excited state. As seen in the Supplementary Table 2 , the first excited state energies and optical transitions shift by ~20 nm to lower energies. The energies are calculated for a neutral dimer in a configuration corresponding to the optimized mixed dimer to account for the rapid excited state formation on charge recombination. The excited state stabilization (lowering of the excited state energy) decreases the rate of the transformation into the excimer state because the process is energetically less favorable. As a result, an increasing part of the energy is emitted from the van der Waals dimer itself and leads to the appearance of the type I spectra ( Fig. 4b ). The model can also account for the broad spectral distribution of type I and spectral dynamics in EL. The interactions between fluorene units located on different parts of the same chain (intramolecular interchain interactions) are determined by the distance and orientation of the chains. The inherent conformational variety of the BDOH-PF chains causes a distribution of the dimer coupling parameters, which results in a distribution of the transition energies and consequently in the distribution of the EL spectra. Conformational dynamics of the chains leads to temporal variations of the dimer coupling parameters and these variations cause the observed EL spectral jumps. An energetically optimal conformation corresponds to the equilibrium observed in the distribution of EL spectral jumps ( Fig. 2h ). Repeated excitation of an energetically unstable dimer tends to produce conformational change that would optimize the energy and cause a spectral jump towards the equilibrium. The most appealing point of the above model is that it would unify in one scheme the different types of emission observed in polyfluorene. We note, however, that an alternative model that would ascribe the type I spectra to the emission of the ground-state aggregates and the type II to the emission of the keto defects is also plausible. The DFT calculation results can be used for such model but the scheme of Fig. 4 would no longer be applicable. The spectral jumps between the type I and type II spectra would reflect conformational changes between states in which the charges are trapped and recombine on the keto defects (type II spectra) and states in which the charges do not reach the defect and are trapped on a fluorene unit of the chain and form the stable ground-state dimer with a neighboring chain (type I spectra). Local chain conformation would be likely the decisive factor in this model as well. We also note that very recently Adachi et al . observed PL from trap states in single chains of poly(9,9-dioctylfluorene) [40] that shows spectra resembling the shape and frequency distribution of the type I observed in PL here. In conclusion, the observed variety of the single-chain EL spectra and the spectral dynamics reflect the complex and rich nature of the photophysics behind the EL process. In addition to the well documented emission from keto defects we found a wide distribution of EL spectra and proposed a mechanism based on a formation and stabilization of ground-state inter-chain aggregates. We note that in bulk EL devices, polyfluorenes with PEO sidechains such as BDOH-PF tend to show much stronger green band emission than polyfluorenes with alkyl sidechains. In the future it will be important to design experiments that would enable to measure on single-chain level the photophysics behind the green EL band of the alkyl-substituted polyfluorenes to shed light on the origin of the differences. Also, it will be interesting to conduct the single-chain EL experiments on other conjugated polymers, such as derivatives of PPV with PEO sidechains, to see if the phenomena found in this work are common to EL of other semiconducting polymers. The results presented in this work are likely to have impact in the field of photophysics of polyfluorenes, and have implications for the material design as well. Materials and sample preparation Poly[9,9-bis(3,6-dioxaheptyl)-fluorene-2,7-diyl] (BDOH-PF) synthesis. The monomer, 2,7-dibromo-9,9-bis(3,6-dioxaheptyl) fluorene was synthesized following ref. 7 . Polymerization was carried out using Yamamoto coupling mainly according to ref. 41 . The product was characterized by 1H nuclear magnetic resonance, ultraviolet-visible absorption and fluorescence spectroscopy. The molecular weight was determined by GPC using a polystyrene standard and THF solvent. The M n was 9,950, M w was 18,600 and the polydispersity index was 1.87. The BC PEO m - b -PMA(Chal) n and the corresponding homopolymers PEO 114 and PMA(Chal) 50 were synthesized mainly using standard methods as described before [30] . BDOH-PF-doped BC films were facbricated by first preparing a 1 wt% chloroform solution of the BC into which small amount of BDOH-PF was added to the final concentrations of 2 × 10 −8 or 2 × 10 −10 M (corresponding to the respective densities of 1 chain per cylinder or 1 chain per 100 cylinders in the phase-separated film). A quantity of 100 μl of the solution was spin coated on cleaned microscope cover slips at 3,000 r.p.m. for 30 s. To obtain hexagonally arranged PEO cylindrical domains, the hybrid films were annealed in vacuum at 90 °C for 2 h. The thickness of the hybrid films was 70 nm as determined using a surface profiler (Veeco, Dektak). Characterization Atomic force microscopy was carried out using Asylum Technology MFP-3D module in tapping mode with an AC240TS-C3 cantilever (Olympus). Transmission electron microscopy experiments were done using a JEM-2100F (JEOL) microscope with BC films prepared on a freshly cleaved mica substrate. The substrate was subsequently immersed in water, the BC film was floated on the water surface and picked up with a Cu grid. The film was stained with RuO 4 to enhance a contrast between PEO and PMA(Chal) microdomains. Bulk PL and EL spectra were measured using a commercial spectrofluorometer. Light-emitting device fabrication Microscope cover glass slips (22 mm × 22 mm, 0.15 mm in thickness) were custom coated via sputtering with ITO (56.2 nm, 100 Ω sq −1 , Geomatec). After electrode pattern etching using a mixture of nitric acid and hydrochloric acid, the substrates were ultrasonically cleaned with acetone, isopropanol and methanol, dried by nitrogen gas and cleaned by a ultraviolet–ozone cleaner. To fabricate the OLEDs, a 40 nm hole injecting layer of poly(3,4-ethylenedioxythiophene) poly(styrenesulfonate) (PEDOT:PSS, Clevios P AI4083, H. C. Starck) was first spin coated on the ITO (4,000 r.p.m., 40 s) and baked at 200 °C for 5 min. The doped BC film of 70 nm thickness was prepared as described above. Finally, an Al electrode (100 nm) was deposited via evaporation. A reference sample for bulk EL experiment was prepared using commercially available polyfluorene with PEO sidechains, ADS160BE (American Dye Source). Neat 70 nm film of ADS160BE was spin coated on the PEDOT:PSS layer and covered with the Al electrode. Single-molecule spectroscopy The EL and PL experiments were carried out on an inverted fluorescence microscope (Olympus IX 71) using oil-immersion objective lens (Olympus UPlanFLN100xO2, N.A. 1.3). The PL was excited with a 375 nm laser (Pico Quant) at 0.6 W cm −2 of excitation power. The emission was dispersed using an imaging spectrograph (Bunkou Keiki CLP-50, 0.5 nm resolution) and detected with an electron multiplication CCD camera (Andor iXon) with typical integration times of 0.1 s for the images and 0.5 s for the spectra and gain of 300. All experiments were done in air at ambient conditions. DFT calculations Multiple initial configurations (>20) for the ground-state dimers were randomly generated and selected for the neutral dimer and for the mixed dimer composed of a neutral fluorene monomer and fluorene cation or anion. Examples of four such energetically most stable configurations (both parallel, D1, and antiparallel, D2–D4) are presented in Supplementary Table 1 . The initial configurations were fully optimized by the long-range corrected density functional including empirical dispersion (ωB97X-D) [42] with the 6-311G (d,p) basis set [43] , [44] . The stationary structures were confirmed by all positive harmonic frequencies. The relevant singlet excited states were characterized by time-dependent DFT [45] . For the interorbital transitions in the mixed dimers ( Supplementary Table 2 ), the ground-state configurations were at first optimized for the neutral—cation or neutral—anion pairs. The ionic counterparts were then replaced by a neutral fluorene and the transition was calculated without changing the mixed dimer configuration. The calculations were carried out using the Gaussian 09 program package [46] . Most of the above calculations were performed on fluorene with methyl groups at the 9,9 positions (Me-fluorene). Control calculations on selected configurations of the dimers were carried on fluorene with the methyl groups replaced by ethylene oxide groups (EO-fluorene) to examine the effect of the bulky sidechains on the dimer formation. How to cite this article : Honmou, Y. et al . Single-molecule electroluminescence and photoluminescence of polyfluorene unveils the photophysics behind the green emission band. Nat. Commun. doi: 5:4666 10.1038/ncomms5666 (2014).